Flexible indium–gallium–zinc–oxide Schottky diode operating beyond 2.45 GHz Mechanically flexible mobile phones have been long anticipated due to the rapid development of thin-film electronics in the last couple of decades. However, to date, no such phone has been developed, largely due to a lack of flexible electronic components that are fast enough for the required wireless communications, in particular the speed-demanding front-end rectifiers. Here Schottky diodes based on amorphous indium–gallium–zinc–oxide (IGZO) are fabricated on flexible plastic substrates. Using suitable radio-frequency mesa structures, a range of IGZO thicknesses and diode sizes have been studied. The results have revealed an unexpected dependence of the diode speed on the IGZO thickness. The findings enable the best optimized flexible diodes to reach 6.3 GHz at zero bias, which is beyond the critical benchmark speed of 2.45 GHz to satisfy the principal frequency bands of smart phones such as those for cellular communication, Bluetooth, Wi-Fi and global satellite positioning. Since wireless radio transmissions were first achieved in the 1880s, telecommunications have evolved to the point where instant global communication is a daily reality, currently contributing more than a trillion dollars to the world economy per year [1] . Consumer demands for higher-performance, more fashionable mobile phones are now unprecedented. Mechanically flexible mobile phones in particular have long been envisaged in the recent rapid development of thin-film electronics. If these visions are realized, such wearable electronics could transform a range of electronic gadget concepts. Among the available flexible semiconductor films, indium–gallium–zinc–oxide (IGZO) has shown perhaps the most commercial potential due to its high electron mobility and possibility of low-temperature film deposition on plastic substrates [2] , [3] , [4] , [5] , [6] . It has already seen rapid adoption as the channel material in backplane driver transistors in some newest flat-panel displays, where a transistor speed of 200 Hz suffices [7] , [8] . In cellular phone communications, transistors are mostly used in logic circuits, which may work at a low clock frequency. The earliest mobile phone processors were typically clocked at a few megahertz [9] . However, the front-end rectifiers must always operate at the transmission microwave frequencies: 935 MHz to 1.88 GHz for cellular communications, around 2.4 GHz for typical IEEE 802.11b/g/n Wi-Fi channels and Bluetooth, 1.58542 and 1.2276 GHz for global satellite positioning, 3.8 GHz for highest 4G long-term evolution (LTE) band and even 5 GHz for the newest 802.11a/h/j/n/ac Wi-Fi channels. There have been highly desirable efforts to develop high-speed Schottky diodes based on metal-oxide semiconductors [10] , organic semiconductors [11] , [12] , [13] , [14] and conventional semiconductors [15] , [16] , [17] . Most of these were on glass substrates, for example, pentacene and C 60 pin diodes working as rectifiers up to 300 MHz [18] ; organic pentacene Schottky diodes operating up to 870 MHz [19] ; diodes based on C 60 and tungsten oxide showing a cut-off frequency of 800 MHz [20] . However, these devices required high-temperature process steps and hence could not be made on plastic substrates. Moreover, these achieve speeds are yet well below 2.45 GHz. So far, the work on flexible substrates is very limited, mainly including polythiophene-based Schottky diodes with a cut-off frequency of 14 MHz [11] , polytriarylamine-based devices with a cut-off frequency of 10 MHz [13] and pentacene-zinc oxide-based diodes with a cut-off frequency of 15 MHz [14] . The frequency limitation of flexible organic diodes restricts their high-speed applications. Conventional semiconductor membranes and particles are another option for active layers in flexible diodes. By transferring single crystalline silicon [15] and germanium [16] membranes on flexible substrates, the diodes demonstrated frequency responses up to 30 GHz and 10 GHz, respectively. The flexible Schottky diodes based on crystalline silicon micro-particles [17] also obtained a cut-off frequency of 1.6 GHz. However, due to the material and process complexity and costs, such technologies are yet to prove commercially viable for flexible electronics. Metal-oxide semiconductors, on the other hand, have already been incorporated into flexible electronics in both academia and industry [7] , [8] , [21] , [22] . To date, most research on metal-oxide semiconductors has focused on thin-film transistors (TFTs) [7] , [8] , [21] , [22] , [23] , and little has been reported on diodes [24] , [25] , [26] , [27] , [28] , [29] , [30] . The recent progresses on high-speed IGZO Schottky diodes including 900 MHz in 2012 (ref. 25 ), 1.8 GHz in 2013 (ref. 26 ) and 3 GHz in 2014 (ref. 27 ), but these were all made on glass substrate using high-temperature annealing processes and hence not applicable to flexible substrates. To the best of our knowledge, the highest frequency obtained on plastic substrates was 27 MHz by IGZO-Cu 2 O diodes [10] . To date, no flexible metal-oxide diodes, to our knowledge, have been able to reach the benchmark speed of 2.45 GHz. In this work, we demonstrate what to our knowledge is the first flexible IGZO Schottky diode fabricated at room temperature and operating beyond 5 GHz without any post-treatment. First, we fabricate Schottky diodes with different IGZO layer thicknesses, and analyse their current–voltage ( J – V ) and capacitance–voltage ( C – V ) characteristics. Second, the intrinsic and extrinsic components that determine the diode cut-off frequencies are extracted from the S-parameter measurements. Based on the relationship between series resistance and capacitance, we provide two methods to further improve the diode speed. Finally, flexible thin-film IGZO Schottky diodes with suitable radio-frequency (RF) mesas are fabricated, and a single-stage rectifier on a polyethylene terephthalate (PET) substrate is demonstrated at frequencies up to 3 GHz. IGZO Schottky diodes on glass substrates For the ease of fabrication and testing, we first use glass substrates to study the effects of some key parameters on the device including direct current (DC) and high-frequency performance. 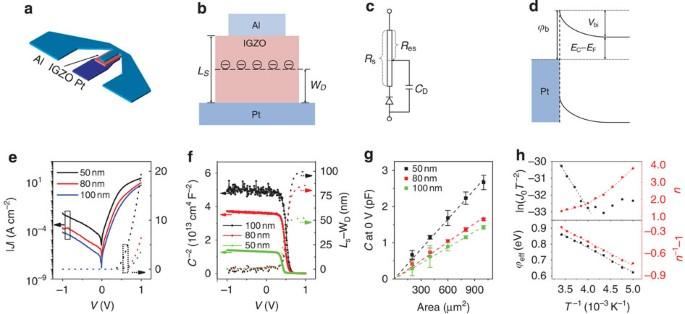Figure 1: DC properties of IGZO Schottky diodes on glass substrate. (a) Structure of the IGZO Schottky diode. The device consists of a 50-nm-thick Pt layer (dark blue), an IGZO layer (red) with a thickness of 50, 80 or 100 nm and an Al electrode (light blue). (b) Cross-section structure of the diode.LSrepresents the thickness of the IGZO layer andWDis the depletion width caused by the Schottky barrier. (c) Equivalent circuit of the IGZO Schottky diode.Rsis the series resistance including the bulk resistance of IGZO and the ohmic contact resistance.Resis the effective series resistance in the rectifier circuit, which is due to the depletion width.CDis the capacitance caused by the depletion layer. (d) Band diagram of the Schottky barrier between IGZO and Pt. The barrier height can be obtained either fromJ–VorC–Vcharacteristics. (e)J–Vcharacteristics of the Schottky diodes with different IGZO thicknesses from 50 to 100 nm. (f) Solid lines represent theC–Vcurves, using which the built-in voltage and background carrier density can be obtained. The dashed lines show the thickness of IGZO layer, which contributes toResas a function of the applied voltage. (g) Capacitance of devices with different sizes and thicknesses under 0 V bias with error bars depicting s.d. In total, we have fabricated five devices under each condition in each of the two rounds of fabrications. (h) Richardson plot and temperature dependency values ofϕeff,nandn−1−1. Figure 1a shows the structure of the IGZO Schottky diode with a vertical design. By adopting the coplanar waveguide and mesa structure, low signal losses at high frequency can be achieved, this also serves to reduce the fringe capacitance and the possibility of breakdown [31] . An aluminium (Al) electrode is used here as the ohmic contact because the work function of Al is only 4.2 eV and the contact resistance between Al and IGZO is known to be quite low [32] . A platinum (Pt) electrode is chosen as the Schottky contact due to its high work function of 5.4 eV [22] . The overlapping region between the two electrodes determines the effective area of the diode. By changing the size of Al ohmic contacts through photolithography, devices with different active areas from 20 × 10 to 20 × 50 μm 2 are obtained. Figure 1b shows the cross-section schematic of the IGZO diodes. Three different IGZO thicknesses have been investigated, that is, L S =50, 80 and 100 nm. In Fig. 1b , W D denotes the depletion depth caused by the bending of the conduction band in the IGZO. The equivalent circuit of the diode is shown in Fig. 1c where R s is the series resistance, comprised of the bulk resistance of the IGZO layer and the ohmic contact resistance from the Al contacts. However, to describe the high-frequency behaviour, the effective series resistance, R es , is introduced. It is obtained from the series resistance R s minus the resistance of the depletion region. This is because under a forward bias, the depletion capacitance is only in series with a part of the series resistance R s , that is, R es , as shown in Fig. 1c . It is the effective series resistance R es that is the main factor in determining the high-frequency performance of the diode. Figure 1d shows the band diagram of the Pt-IGZO Schottky junction, where ϕ b is the barrier height, V bi is the built-in voltage, and E C − E F describes the energy gap between the conduction band and Fermi level. Figure 1: DC properties of IGZO Schottky diodes on glass substrate. ( a ) Structure of the IGZO Schottky diode. The device consists of a 50-nm-thick Pt layer (dark blue), an IGZO layer (red) with a thickness of 50, 80 or 100 nm and an Al electrode (light blue). ( b ) Cross-section structure of the diode. L S represents the thickness of the IGZO layer and W D is the depletion width caused by the Schottky barrier. ( c ) Equivalent circuit of the IGZO Schottky diode. R s is the series resistance including the bulk resistance of IGZO and the ohmic contact resistance. R es is the effective series resistance in the rectifier circuit, which is due to the depletion width. C D is the capacitance caused by the depletion layer. ( d ) Band diagram of the Schottky barrier between IGZO and Pt. The barrier height can be obtained either from J – V or C – V characteristics. ( e ) J – V characteristics of the Schottky diodes with different IGZO thicknesses from 50 to 100 nm. ( f ) Solid lines represent the C – V curves, using which the built-in voltage and background carrier density can be obtained. The dashed lines show the thickness of IGZO layer, which contributes to R es as a function of the applied voltage. ( g ) Capacitance of devices with different sizes and thicknesses under 0 V bias with error bars depicting s.d. In total, we have fabricated five devices under each condition in each of the two rounds of fabrications. ( h ) Richardson plot and temperature dependency values of ϕ eff , n and n −1 −1. Full size image In this work, the Schottky diode performance is optimized by testing different IGZO layer thicknesses and oxygen/argon ratios during the sputtering deposition process of the IGZO film. It is widely accepted that in IGZO TFTs, an excess oxygen content will degrade the film stability and mobility [33] . For the IGZO Schottky diodes in our experiment, the thickness of IGZO is no more than 100 nm. At low-voltage biases, the diode performance is limited by the Schottky junction barrier instead of the IGZO mobility. The extra oxygen during the IGZO deposition is used to passivate the dangling bonds at the Schottky interface to reduce the Fermi level pinning effect [30] (shown in Supplementary Fig. 1 and Supplementary Table 1 ). At high biases, the current is limited by the series resistance, which is related to the IGZO mobility. It is found in this work that 3% oxygen during the deposition results in a good compromise with a high quality Schottky barrier and a relatively low series resistance. The J – V characteristics of the diodes with different IGZO thicknesses are shown in Fig. 1e . The diode with a 50 nm IGZO layer exhibits the highest current, while the device with a 100 nm IGZO layer shows the highest rectification ratio. 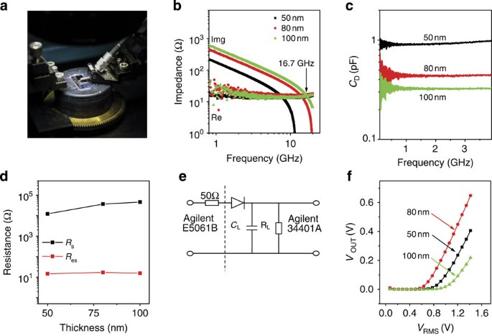Figure 2: High-frequency properties of IGZO Schottky diodes on glass substrates. (a) Photograph of the sample and RF coplanar probe used for the high-frequency characterizations. (b) Resistance and reactance of the 20 × 20 μm2IGZO Schottky diodes at different frequencies. The thickness of the IGZO layer varies from 50 to 100 nm. (c) Capacitance of the IGZO Schottky diodes with different thicknesses as a function of the frequency. (d) Total series resistanceRsand effective series resistanceResas a function of the IGZO layer thickness. (e) Circuit diagram of the single-stage rectifier.RLstands for the load resistor andCLrepresents the load capacitor. (f) Rectification properties of the 20 × 40 μm2diodes with different IGZO layer thicknesses at 1 GHz. Detailed analyses are summarized in Supplementary Table 2 and Supplementary Fig. 2 . At an applied voltage of 1 V, the diode with a 50-nm-thick IGZO layer between the Pt and Al contacts exhibited a current density of 20 A cm −2 giving a total DC resistance of 0.05 Ω cm 2 . When the IGZO layer becomes thicker, the current density drops. At an applied voltage of 1 V, the total resistance for the devices with IGZO thicknesses of 80 nm and 100 nm are 0.15 Ω cm 2 and 0.26 Ω cm 2 respectively. This shows that the series resistance has a sensitive dependence on the thickness of IGZO layer. Given that the effective Richardson constant of IGZO is 41 A cm 2 K 2 and based on the thermionic emission theory [22] , [34] , [35] , the extracted barrier heights are 0.79 eV, 0.73 eV and 0.65 eV for the diodes with 100 nm, 80 nm, and 50 nm IGZO layer, respectively (fitting is shown in Supplementary Fig. 3 ). It is not clear why a thicker IGZO layer results in a higher Schottky barrier, perhaps it is due to the electrode evaporation process in vacuum [2] , [28] . Pt-IGZO Schottky barrier is sensitive to the oxygen content at the interface [30] . During the evaporation process, oxygen may escape from the IGZO layer, causing oxygen deficiency. Such defects are responsible for the Fermi level pinning, resulting in lower barrier heights and built-in voltages. Doping from the top electrode may also contribute to lowering the series resistance (shown in Supplementary Fig. 4 ). The C – V characteristics of the devices with different IGZO layer thicknesses are shown in Fig. 1f . At low forward biases, the capacitance remains almost constant, suggesting that the IGZO layer is fully depleted in each of the devices. Using C=ɛ 0 ɛ r / L S , where ɛ 0 is the vacuum permittivity, the relative dielectric constant of IGZO, ɛ r , is found to be 16. The dotted line represents the thickness of IGZO, which contributes to the effective series resistance R es . It shows that at ∼ 0.7 V, the depletion width becomes negligible when compared with the thickness of the IGZO layer in all the three devices, that is, L S » W D . From the C −2 curves in Fig. 1f , the built-in voltage, V bi , and the background charge density, N bg , can be extracted. From the series resistance obtained from the J – V characteristics of an 80-nm-thick IGZO Schottky diode, the free carrier density is 3.33 × 10 13 cm −3 , which is orders of magnitude lower than the background doping density, and 5.01 × 10 16 cm −3 due to the subgap traps in IGZO [12] . The energy-dispersive X-ray spectroscopy (EDX) measurement suggests that In/Ga/Zn ratio is 4.2:4.4:2.0 as shown in Supplementary Fig. 5 . According to the study conducted by Olziersky et al. [36] , the moderate In/Ga atom ratio of 0.95 should yield a reasonably high carrier mobility. We have therefore assumed that the mobility of IGZO is 10 cm 2 V −1 s −1 (roughly the mobility value obtained from TFTs based on similar IGZO material [22] , [28] , [30] ). Figure 1d shows that the barrier height can be obtained from the sum of V bi and E C −E F . Based on Supplementary Note 1 , ( E C −E F ) is found to be 0.308 eV and hence the barrier height from the C – V plot is 0.864 eV. It is higher than the barrier height from J – V characteristics, which is most likely because of the imperfect uniformity of the Schottky junction [22] . In Fig. 1g , the capacitance of the IGZO Schottky diode at 0 V bias is proportional to A / L S , where A is the area of the device. It shows that there are two ways to reduce the device capacitance, namely by shrinking the size of the device and by increasing the thickness of IGZO layer. Figure 1h shows the temperature-dependent values of the diode derived from the J – V characteristics. The Richardson plot suggests that the current transport is governed by thermionic emission since the diffusion transport is less sensitive to temperature [37] . The large deviation at low temperatures can be explained by the barrier height fluctuation model, that is, the barrier height follows a Gaussian distribution, ϕ eff =ϕ m – qσ 2 /(2 k B T ), where ϕ eff is the effective barrier height, ϕ m is the mean barrier height and σ is the s.d. [37] . It is found that for the diode with an IGZO thickness of 80 nm and a diameter of 1 mm, the mean barrier height is 1.40 eV with a s.d. of 0.17 eV. Furthermore, ( n −1 −1) has a linear dependency with T −1 , which implies the inhomogeneities in the barrier height. The cause of the barrier fluctuation is considered to be a consequence of IGZO grain boundaries, oxygen deficiency and different Pt crystalline orientations [22] . A comparison of background doping density and free carrier concentration highlights an interesting difference between IGZO and traditional covalent semiconductors, namely, not all ionized atoms in IGZO contribute free carriers; this discrepancy can be attributed to subgap traps [30] . Given the direct dependency of the C – V relationship on the background doping concentration, it is expected that the C – V barrier height shall be lower than the mean barrier height obtained by the low-temperature measurement. High-frequency properties on glass substrates To study the high-frequency properties of the diodes, it is necessary to analyse the S-parameter of the device to extract the capacitive and resistive components of the diodes. Figure 2a shows a photograph of the sample and RF coplanar probe used for the high-frequency characterizations. Figure 2b presents that the effective series resistance R es and reactance of the diode at different frequencies determined from the S-parameter at zero bias. As shown in Fig. 2d , the obtained R es is very different from the total series resistance R s that is determined from the J – V curves. While R s varies much more significantly, R es is virtually constant for different IGZO thicknesses. This confirms that when the IGZO layer is fully depleted, the ohmic contact resistance is considered as the sole contributor to the series resistance. Figure 2c shows that the capacitive components of devices remain fairly constant as a function of the frequency, and the capacitive values are in good agreement with the previous C – V measurement results. Figure 2: High-frequency properties of IGZO Schottky diodes on glass substrates. ( a ) Photograph of the sample and RF coplanar probe used for the high-frequency characterizations. ( b ) Resistance and reactance of the 20 × 20 μm 2 IGZO Schottky diodes at different frequencies. The thickness of the IGZO layer varies from 50 to 100 nm. ( c ) Capacitance of the IGZO Schottky diodes with different thicknesses as a function of the frequency. ( d ) Total series resistance R s and effective series resistance R es as a function of the IGZO layer thickness. ( e ) Circuit diagram of the single-stage rectifier. R L stands for the load resistor and C L represents the load capacitor. ( f ) Rectification properties of the 20 × 40 μm 2 diodes with different IGZO layer thicknesses at 1 GHz. Full size image As illustrated in Fig. 1c , the cut-off frequency of the diode should be determined by R es and the capacitance, f =1/2 πR es C D . Since R es is fairly constant in all devices with different IGZO thicknesses, the results might seemingly suggest that the diode with 100-nm-thick IGZO should have the lowest capacitance and hence the best high-frequency performance. To test this, a single-stage rectifier measurement set-up shown in Fig. 2e is used, which involves a 100 nF load capacitor C L and a 1 MΩ load resistor R L . The input signal is generated by Agilent E5061B ENA network analyser and the rectified DC output is measured by Agilent 34401 A voltage meter. Figure 2f plots the dependence of the output voltage as a function of the root mean square (r.m.s) voltage of the input RF signal at 1 GHz, the result is entirely unexpected because the 100 nm diode actually exhibits the worst performance. To understand this, we refer to the set-up in Fig. 2e . On the application of an alternating current (AC) signal, the diode is negatively biased during most of a period of the AC signal due to the positive DC voltage accumulated over the load capacitor. However, the capacitor is only charged during the short duration in each period when the diode is positively biased. For instance, the peak input voltage when V r.m.s =1 V is 1.41 V, at which the 80 nm diode produces a DC output of about 0.3 V, meaning the diode is forward biased at 1.1 V. At such a large forward bias, the IGZO depletion layer thickness becomes small, meaning that part of the IGZO layer shall contribute to the effective series resistance R es . Preliminary results have indicated that R s of the 100 nm IGZO device is about five times that of the 50 nm diode at 1 V, and hence seriously reduced its ability to produce a large rectified output voltage despite having the lowest capacitance. We thus conclude that the hypothesis—the thicker IGZO layer the better the high-frequency performance—is only valid below a critical value. Besides, the output voltage is measured across the 1 MΩ load resistor. As the IGZO thickness increases, the series resistance increases and results in a smaller voltage drop on the load resistor and a decrease in the rectified voltage. With this, we choose 80 nm as the IGZO layer thickness for the following work on flexible substrate. Flexible Schottky diodes and GHz operations Having optimized the diode properties on glass substrate, we have fabricated devices on Dupont flexible PET films using the same lithography steps. The devices are bendable as illustrated in Fig. 3a . The J – V characteristics are shown in Fig. 3b , which yields an ideality factor of 2.1 and a barrier height of 0.51 eV. From the C – V curve in Fig. 3c , the built-in voltage is found to be 0.45 V. As expected, compared with the diodes fabricated on glass substrates under the same condition, the performance of the flexible devices is more affected by the inhomogeneous barrier height caused by the uneven substrate surface. 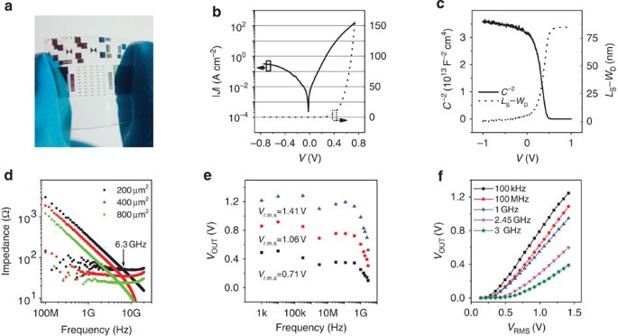Figure 3: Flexible diodes and high-frequency operations. (a) Photograph of flexible IGZO Schottky diodes. (b)J–Vcharacteristics of the flexible diode with an 80 nm IGZO layer. (c) Capacitance and depletion width of the diode at different DC voltages. (d) Impedance of the flexible IGZO Schottky diodes as a function of frequency. (e) Output DC voltage as a function of the input signal frequency at different input signal strengths. (f) Output DC voltage as a function of the input RF signal r.m.s voltage at different frequencies. Figure 3d shows the curves of reactance and resistance versus frequency, which are obtained from the S-parameters of the devices with different active areas. Since the cut-off frequency is given by the intersection of resistance and reactance curves, for the devices with an area of 200 μm 2 , the cut-off frequency is found to be 6.3 GHz. This is the highest achieved in our studies. The cut-off frequency of the devices with an area of 400 and 800 μm 2 is also higher than 5 GHz. Such zero-bias cut-off frequency is commonly regarded as the intrinsic speed of the diodes. When the diode is used in practical applications, such as a rectifying circuit, load resistance, impedance matching and losses from the transmissions will need to be considered. Figure 3: Flexible diodes and high-frequency operations. ( a ) Photograph of flexible IGZO Schottky diodes. ( b ) J – V characteristics of the flexible diode with an 80 nm IGZO layer. ( c ) Capacitance and depletion width of the diode at different DC voltages. ( d ) Impedance of the flexible IGZO Schottky diodes as a function of frequency. ( e ) Output DC voltage as a function of the input signal frequency at different input signal strengths. ( f ) Output DC voltage as a function of the input RF signal r.m.s voltage at different frequencies. Full size image The single-stage rectifier circuit is used again to test the diode performance at high frequencies. Figure 3e shows the output voltage versus frequency at different input signal strengths. Figure 3f plots the output DC voltage as a function of the input RF signal voltage at different frequencies. When the frequency of the input signal increases, the output voltage starts to drop. Even though the output reduces with the frequency, at 2.45 GHz the rectified voltage is measured to be 0.6 V for an input r.m.s voltage of 1.41 V. We note that this is at the maximum output of our signal source, and the diode output can certainly increase with a stronger input signal. So far, we have demonstrated that flexible Pt-IGZO Schottky diodes exhibit an intrinsic cut-off frequency of 6.3 GHz. It is of course possible to adopt the multistage rectifier circuits to double or triple the output voltage as often used in many RFID circuits [38] . As such, the Pt-IGZO diodes may be suitable as the front-end rectifier and power supply in a variety of low-voltage operation devices. To further increase the device performance, some treatments can be adopted for the IGZO Schottky diodes. As mentioned in several studies before [22] , [30] , a post-annealing process can improve the diode barrier height and ideality factor. Fast laser annealing has been successfully demonstrated to treat IGZO TFTs on flexible substrate without heating the substrate beyond the glass transition temperature [5] . Considering that the diode is highly negatively biased in practical rectifier circuits, the diode breakdown voltage is an important parameter. In Supplementary Fig. 6 , the diode with the same fabrication process in our experiment exhibits excellent reverse current characteristics, showing a negative breakdown voltage >10 V. Also, the IGZO Schottky diodes show good air stability, and almost no degradation is observed after 30-day exposure in air as illustrated in Supplementary Fig. 7 . In the single-stage rectifier circuit, the output performance is not only related to the intrinsic cut-off frequency of the diode, but is also influenced by the quality of the load resistance and impedance matching. Due to the frequency-dependent impedance of the diode, it is impossible to avoid the signal reflection and power loss at all frequencies. However, in most application scenarios, the circuit only operates in a certain frequency band. Thus, the system can be specifically designed to maximize power transfer and output within a fairly narrow band. Regarding the perspectives of flexible smart phones, the mechanical flexibility may well attract customers through new user experiences, fashion and style rather than the data processing capacity. Although silicon chips currently dominate, Nokia’s early personal digital assistant, Nokia 9000 Communicator, has an i386 CPU containing ∼ 300,000 transistors. In comparison, the recently developed IGZO-TFT-driven 14′′ display by Fujitsu has a 3,200 × 1,800 resolution, meaning that the display backplane driver contains millions of transistors. Furthermore, the recently developed p-type SnO with good mobility and stability has already enabled successful CMOS logic gates [39] . In terms of transistor speed, Yin et al. [40] demonstrated IGZO ring oscillators at 106.5 MHz with a 0.5 μm channel length. By reducing the device size to the current Silicon technology node of 14 nm, IGZO circuits can well operate at gigahertz frequencies. In summary, we have reported the first flexible IGZO Schottky diodes with cut-off frequency up to 6.3 GHz. By analysing the J – V and C – V characteristics, a high-frequency model is proposed. Surprisingly, the hypothesis that the thicker IGZO layer the better the high-frequency performance is found to be invalid in the experiments and our finding is discussed in terms of the series resistance and capacitance under different biases. By combining such GHz IGZO diodes with less speed-demanding TFTs, a range of flexible microwave circuits and possibly mobile phones may be constructed. Device fabrication Corning 7059 glass and Dupont Melinex PET film were used as substrates in this experiment. Before the fabrication, the substrates were degreased by supersonic cleaning in deionized water, acetone and methanol, then dried with nitrogen and placed in UV/Ozone chamber for 30 min. Pt electrodes (50-nm-thick) were deposited by RF sputtering at 80 W in pure argon. And subsequently IGZO (In/Ga/Zn=1:1:1, Lesker) was sputtered at 80 W in argon with 3% oxygen at 0.5 Pa. The Al electrodes were formed by using thermal evaporation. Patterns were defined by photolithography with standard processes. All devices were fabricated and tested at room temperature without any thermal annealing process. Measurements The J – V characteristics were made using Agilent E5260B Semiconductor analyser at room temperature in dark. Agilent E4980A LCR meter was used to measure the capacitance of IGZO Schottky diodes. The DC output of the IGZO Schottky diodes was measured by Agilent 34401 A digital multi-meter. The coupling to the device was through RF probes (GGB Industries Inc.) and the AC signal was generated by Agilent E5061B network analyser. The S-parameters were measured by Agilent PNA-X N5247A network analyser after calibration. The EDX spectroscopy was performed by an FEI Nova NanoSEM 450 scanning electron microscope with an Oxford Instrument X-Max N Silicon Drift Detector. The measurements were performed at 20 keV with a scan area of 51 × 34 μm. The In–L, Ga–K and Zn–K peaks were selected for the analyses. How to cite this article : Zhang, J. et al. Flexible indium gallium zinc oxide Schottky diode operating beyond 2.45 GHz. Nat. Commun. 6:7561 doi: 10.1038/ncomms8561 (2015).